IL-10 inhibits neuraminidase-activated TGF-β and facilitates Th1 phenotype during early phase of infection Th1 cells control their activity by producing regulatory IL-10. Here we report that Th1 cell-derived IL-10 facilitates their expansion and, in addition, augments Th1 cell production of IFN-γ, TNF-α and IL-2 during the early phase of influenza. In our antigen-specific mouse experimental system, influenza haemagglutinin-specific CD4 + T cells respond to infection with the induction of T-bet, and produce both IFN-γ and IL-10. In the early phase of infection, an abundance of viral neuraminidase causes TGF-β activation of haemagglutinin-specific CD4 + T cells. CD4 + T-cell-derived IL-10 inhibits neuraminidase-driven TGF-β activation and counteracts the virus-mediated immune suppression. As the host eradicates the virus, neuraminidase activity wanes and IL-10 receptors are upregulated on CD4 + T cells in the late phase of infection. IL-10 then suppresses immune activation and aids in recovery from infection and inflammation. These results reveal a previously unrecognized function of Th1 cell-derived IL-10 in vivo . The influenza virus attacks millions of people worldwide and causes significant numbers of deaths every year. The potential for morbidity and mortality increases in pandemic years ( http://www.cdc.gov/flu/about/disease/ ). The clinical outcome of an infection depends primarily on the interplay between the virus and the host immune reactions to the infection. The influenza virus uses strategies to circumvent host defenses for the establishment of infection and efficient replication [1] , [2] . The host immune system, on the other hand, responds to limit viral spread, as well as to eradicate the virus [3] , [4] , [5] , [6] , [7] , [8] . Such responses may result in the excessive production of inflammatory cytokines that cause lung injury and damage to the host [3] , [4] , [5] , [6] , [7] , [8] . Upon infection with influenza virus, the host antiviral response is activated with extensive proliferation and robust production of inflammatory cytokines by CD4 + T cells. Viral neuraminidase (NA) cleaves glycosidic bonds of sialic acids on the host cell surface. This cleavage facilitates viral entry and exit from the cells [9] . It also activates latent transforming growth factor (TGF)-β by removing the sialic acids on the N-terminal latency-associated peptide (LAP) [10] . Active TGF-β mediates immune suppression, including regulation of T cells [11] , [12] , [13] , [14] , and contributes to evasion by the pathogen from the immune response [15] , [16] , [17] , [18] . In influenza virus infections, interleukin (IL)-10 is secreted in significant amounts, along with effector inflammatory cytokines [2] , [3] , [4] , [5] , [6] , [19] , [20] . The role of IL-10 in influenza virus infections remains ambiguous. Increased levels of IL-10 have been linked to severe lung inflammation and fatality in human influenza [5] , [7] . In experimental mice, IL-10 seems to aggravate the disease. IL-10 knockout (KO) mice survive better than wild-type (WT) mice upon infection with influenza virus [21] , [22] . However, IL-10 receptor (IL-10R) blockade after 3 days of infection increases mortality with aggravated pulmonary inflammation in mice [19] . IL-10 modulation at different time points in infection generates a difference in outcome from the infection. Perhaps IL-10 plays dissimilar roles in different phases of influenza virus infection. Here we study host immune responses to influenza virus infection through the use of an influenza haemagglutinin (HA) antigen-specific transgenic mouse model [20] . A HA-specific CD4 + T-cell response represents the antigen-specific CD4 + T-cell response to influenza virus infection. CD4 + T-cell activity is essential for harnessing the antibody and the cytotoxic T-cell responses that are critical for viral clearance [23] , [24] , [25] , [26] . In our system, mice received naive HA-specific CD4 + T cells by adoptive transfer with infection of H1N1 influenza virus. HA-specific CD4 + T cells responded to the viral HA with the induction of T-bet, and additionally produced Th1 cytokines and IL-10 (ref. 20 ). The HA-specific Th1 cell-derived IL-10 inhibited influenza NA-activated TGF-β and facilitated production of interferon (IFN)-γ in the Th1 cells during the early phase of infection. The NA activity waned with viral clearance. IL-10 then suppressed immune activation in the absence of viral NA and aided in recovery from inflammation and disease during the late phase of infection. Our findings demonstrate how Th1 cell-derived IL-10 performs to counteract viral immune suppression and augment inflammation during the early phase of influenza virus infection. Influenza virus infection drives an HA-specific Th1 response In our influenza HA antigen-specific mouse model [20] , syngeneic mice received 2.5 × 10 6 naive 6.5 HA-specific CD4 + T cells by adoptive transfer. The recipient mice were infected with 2.5 × 10 3 plaque-forming units (p.f.u.) of the PR8 strain of H1N1 influenza virus on the same day as cell transfer. The infected mice showed disease symptoms, such as ruffled hair, and started to lose weight from day 4 post infection. They continued to decline for ~1 week and then the majority of the mice started to regain weight and recover from the disease. The 6.5 HA-specific CD4 + T cells responded to infection with the production of Th1 cytokines IFN-γ, TNF-α and IL-2, along with increased levels of IL-10 ( Supplementary Fig. 1a ). The majority of IL-10-positive cells secreted IFN-γ as IL-10/IFN-γ double-positive cells ( Supplementary Fig. 1b ). T-bet, the hallmark transcription factor for Th1 cells, was induced in the HA-specific CD4 + T cells as well ( Supplementary Fig. 1c ). NA and active TGF-β release in the early phase of infection Viral NA increases with multiplication of virus during the early phase of infection. NA is known to cause activation of latent TGF-β in the lungs [10] . As most of the cell types possess latent TGF-β, we tested whether viral NA activates TGF-β in 6.5 HA antigen-specific CD4 + T cells. As the virus multiplied (closed bars, Fig. 1a ), the activity of viral NA increased in the 6.5 HA-specific CD4 + T cells of mouse lungs from day 2 to day 4 post infection, as measured by the lectin, peanut agglutinin (PNA), binding (top panels, Fig. 1b ) and LAP staining ( Supplementary Fig. 2 ) on the cell surface. Viral NA cleaved sialic acids on the cell surface and exposed LAP on the membrane. Desialylation resulted in PNA binding on the cell surface. The release of active TGF-β in 6.5 HA-specific CD4 + T cells increased with augmented viral NA activity (top panels, Fig. 1c ), similar to previous reports on TGF-β activation by influenza NA [10] , [27] . Viral NA also desialylated and exposed LAP on the membrane, and activated TGF-β in the HA-specific CD4 + T cells in the draining lymph nodes of the lung (mediastinal lymph nodes, MLN; Supplementary Fig. 2 ). The enzymatic activity of viral NA waned with time and the activity in the lung on day 5 was comparable to those of uninfected control mice with synchronous adoptive transfer of naive 6.5 HA-specific CD4 + T cells. The viral titre declined after day 6 post infection ( Fig. 1a ) and became undetectable on day 11 post infection. 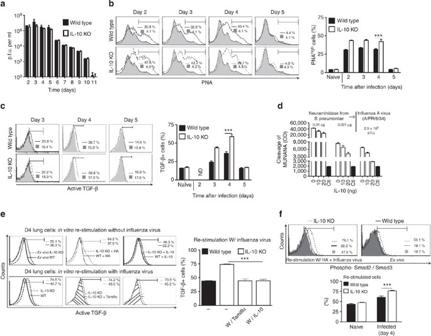Figure 1: IL-10 inhibits influenza NA-driven release of active TGF-β in influenza HA-specific CD4+T cells during the early phase of infection. Naive WT or IL-10 KO HA-specific CD4+T cells were adoptively transferred into WT or IL-10 KO mice, respectively, with 2.5 × 103p.f.u. of influenza virus infection, as described in text. (a) Viral titres in the lungs; (b) surface PNA binding on HA-specific CD4+T cells from lungs on stated days post infection; (c) intracellular active TGF-β levels onex vivoHA-specific CD4+T cells from lungs on stated days post infection. HA-specific CD4+T cells adoptively transferred into naive mice without infection served as the control (grey shades). (d) IL-10-mediated inhibition of NA activity: the dose–response relation between the IL-10 concentration and NA-mediated substrate cleavage. Control (ctl) refers to the background fluorescence of substrate without influenza virus and IL-10. (e) Intracellular active TGF-β in WT and IL-10KO HA-specific CD4+T cells from the lungs on day 4 post infection. Lung cells were analysed after re-stimulation in the absence or presence of influenza virus. (f) Phospho- Smad2/Smad3 levels in WT and IL-10 KO HA-specific CD4+T cells from the lungs on day 4 post infection. Cells were analysed eitherex vivoor afterin vitroculture with influenza virus. Naive HA-specific CD4+T cells from non-infected mice served as the control. Values are mean±s.d. of at least three experiments (ND, not detected;n=6; ***P< 0.0001; two-tailedPvalues for unpairedt-test). Figure 1: IL-10 inhibits influenza NA-driven release of active TGF-β in influenza HA-specific CD4 + T cells during the early phase of infection. Naive WT or IL-10 KO HA-specific CD4 + T cells were adoptively transferred into WT or IL-10 KO mice, respectively, with 2.5 × 10 3 p.f.u. of influenza virus infection, as described in text. ( a ) Viral titres in the lungs; ( b ) surface PNA binding on HA-specific CD4 + T cells from lungs on stated days post infection; ( c ) intracellular active TGF-β levels on ex vivo HA-specific CD4 + T cells from lungs on stated days post infection. HA-specific CD4 + T cells adoptively transferred into naive mice without infection served as the control (grey shades). ( d ) IL-10-mediated inhibition of NA activity: the dose–response relation between the IL-10 concentration and NA-mediated substrate cleavage. Control (ctl) refers to the background fluorescence of substrate without influenza virus and IL-10. ( e ) Intracellular active TGF-β in WT and IL-10KO HA-specific CD4 + T cells from the lungs on day 4 post infection. Lung cells were analysed after re-stimulation in the absence or presence of influenza virus. ( f ) Phospho- Smad2/Smad3 levels in WT and IL-10 KO HA-specific CD4 + T cells from the lungs on day 4 post infection. Cells were analysed either ex vivo or after in vitro culture with influenza virus. Naive HA-specific CD4 + T cells from non-infected mice served as the control. Values are mean±s.d. of at least three experiments (ND, not detected; n =6; *** P < 0.0001; two-tailed P values for unpaired t -test). Full size image IL-10 inhibits early viral NA-driven active TGF-β release Next we tested the impact of the cytokine IL-10 on the enzymatic activity of viral NA. In a chemical assay, IL-10 inhibited the enzymatic action of influenza NA and NA-A of Streptococcus pneumoniae ( Fig. 1d ). IL-10-mediated inhibition of viral NA activity was also evident when the in vivo activity was compared between IL-10-competent and IL-10-deficient mice. We transferred naive IL-10 KO 6.5 HA-specific CD4 + T cells into IL-10 KO mice, similar to the transfer of naive WT 6.5 HA-specific CD4 + T cells into WT mice. When the virus multiplied during the early phase of influenza virus infection in the IL-10 KO mice, viral NA desialylated the surface of IL-10 KO HA-specific CD4 + T cells and caused the release of active TGF-β from day 2 to day 4 post infection, similar to the WT cells in WT mice ( Fig. 1a–c ). However, the IL-10 KO HA-specific CD4 + T cells revealed more desialylation ( Fig. 1b ), more LAP expression and more active TGF-β release compared with the WT HA-specific CD4 + T cells in the lungs and MLN of WT-recipient mice ( Fig. 1b,c,e and Supplementary Fig. 2 ). The viral NA-driven activation of TGF-β was not restricted in the antigen-specific CD4 + T cells in the lungs of influenza virus-infected mice. Flow cytometric analysis revealed elevated active TGF-β level on the lung cells of infected compared with non-infected mice on day 4 post infection. Also, enzyme-linked immunosorbent assay data from the lung lysates of infected mice revealed higher levels of active TGF-β than in the non-infected mice ( Supplementary Fig. 3 ). Active TGF-β levels were higher in the lung lysates of the IL-10 KO mice relative to the WT-infected mice on day 4 post infection ( Supplementary Fig. 3 ). However, the serum levels of TGF-β by enzyme-linked immunosorbent assay were not significantly different among infected or non-infected IL-10 KO or WT mice on day 4 post infection. In vitro re-stimulation with influenza virus increased active TGF-β further by both ex vivo IL-10 KO and WT HA-specific CD4 + T cells on day 4 post infection. Re-stimulation amplified the difference between IL-10KO and WT cells, with more active TGF-β in IL-10 KO relative to WT HA-specific CD4 + T cells ( Fig. 1e ). NA inhibitor Oseltamivir (Tamiflu) reduced active TGF-β in the IL-10 KO HA-specific CD4 + T cells in the re-stimulation of ex vivo cells on day 4 post infection ( Fig. 1e ). Exogenous IL-10 also reduced active TGF-β levels in the IL-10 KO HA-specific CD4 + T cells ( Fig. 1e ). The increased level of active TGF-β caused hyper-activation of downstream signalling in the IL-10 KO HA-specific CD4 + T cells. There was more phosphorylated Smad2/Smad3 in the IL-10 KO HA-specific CD4 + T cells in the lungs of IL-10 KO mice compared with the WT HA-specific CD4 + T cells in the lungs of WT mice on day 4 post infection ( Fig. 1f ). IL-10 facilitates early-phase HA-specific Th1 evolution We compared the immune activation during the early phase of influenza virus infection in the absence or presence of IL-10. We performed an adoptive transfer of naive IL-10 KO 6.5 HA-specific CD4 + T cells into IL-10 KO mice and WT 6.5 HA-specific CD4 + T cells into WT mice. With a total absence of IL-10 in the IL-10 KO adoptive transfer set, activation of HA-specific CD4 + T cells was attenuated compared with the IL-10-competent WT adoptive transfer set. Clonotypic expansion was decreased and both CD44/CD69 upregulation and CD62L downregulation were impeded ( Fig. 2a ). Inflammatory cytokine production, such as IFN-γ, TNF-α, IL-2, IL-6 and IL-17a, was also decreased in the absence of IL-10, except for a transient increase in levels of IL-6 and IL-17a on day 7 ( Fig. 2b ). However, the Th1 polarity was unaltered with IL-10 deficiency, as the induction of T-bet was comparable between HA-specific CD4 + T cells of the IL-10 KO and WT adoptive transfer sets ( Fig. 2c ). The Th1 response kinetics was different in the presence or absence of IL-10. The WT response peaked earlier than that of the IL-10 KO. Impeded activation of IL-10 KO HA-specific CD4 + T cells was associated with less expansion, as revealed by fewer cell divisions in vivo ( Fig. 3a ). Activation-induced cell death was similar between IL-10 KO and WT CD4 + T cells ( Fig. 3b ). Attenuated activation of IL-10 KO HA-specific CD4 + T cells was not due to augmented regulation by regulatory T cells. Both natural (Foxp3 + ) and induced ( Fig. 3c ) regulatory T cells were comparable in amount among IL-10 KO HA-specific CD4 + T cells, WT HA-specific CD4 + T cells and endogenous CD4 + T cells. 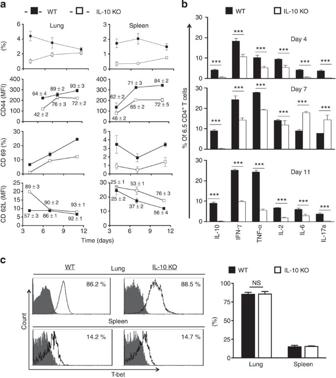Figure 2: Influenza HA-specific CD4+T-cell activation is impeded in the absence of IL-10. Naive WT or IL-10 KO HA-specific CD4+T cells were adoptively transferred into WT or IL-10 KO mice, respectively, with 2.5 × 103p.f.u. of influenza virus infection, as described in text. (a) Activation as revealed by clonotypic expansion and activation marker profiles. Numbers in the panels represent the percentages of CD44highand CD62Llowcells on corresponding days post infection. (b) Activation as revealed by cytokine production of 6.5 CD4+T cells from the lungs on stated days post infection. (c) T-bet expression of HA-specific 6.5 CD4+T cells in the lungs on day 7 post infection. HA-specific CD4+T cells adoptively transferred into naive mice without infection served as the control (filled area). Values are mean±s.d. of at least three experiments (MFI, mean fluorescence intensity;n=6; ***P< 0.0001; *P< 0.01; NS, nonsignificant,P>0.05; two-tailedPvalues for unpairedt-test). Figure 2: Influenza HA-specific CD4 + T-cell activation is impeded in the absence of IL-10. Naive WT or IL-10 KO HA-specific CD4 + T cells were adoptively transferred into WT or IL-10 KO mice, respectively, with 2.5 × 10 3 p.f.u. of influenza virus infection, as described in text. ( a ) Activation as revealed by clonotypic expansion and activation marker profiles. Numbers in the panels represent the percentages of CD44 high and CD62L low cells on corresponding days post infection. ( b ) Activation as revealed by cytokine production of 6.5 CD4 + T cells from the lungs on stated days post infection. ( c ) T-bet expression of HA-specific 6.5 CD4 + T cells in the lungs on day 7 post infection. HA-specific CD4 + T cells adoptively transferred into naive mice without infection served as the control (filled area). Values are mean±s.d. of at least three experiments (MFI, mean fluorescence intensity; n =6; *** P < 0.0001; * P < 0.01; NS, nonsignificant, P >0.05; two-tailed P values for unpaired t -test). 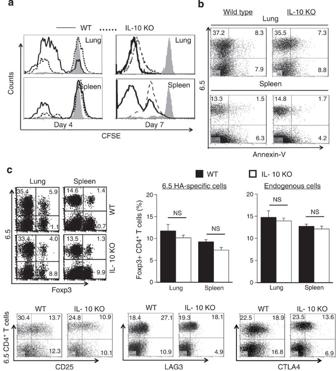Figure 3: Impeded HA-specific CD4+T-cell activation in the absence of IL-10 is not related to increased apoptosis or expanded regulatory T-cell populations. Naive WT or IL-10 KO HA-specific CD4+T cells were adoptively transferred into WT or IL-10 KO mice, respectively, with 2.5 × 103p.f.u. of influenza virus infection, as described in text. (a) CFSE staining profiles of HA-specific 6.5 CD4+T cells on stated days post infection. HA-specific 6.5 CD4+T cells adoptively transferred into naive mice without infection served as the control (grey shades). (b) Annexin-V staining of 6.5+and endogenous CD4+T cells in stated organs on day 7 post infection. (c) Regulatory T-cell populations. Top panels: Foxp3+T cells among 6.5 HA-specific or endogenous CD4+T cells on day 7 post infection. Values are mean±s.d. of at least three experiments;n=6; NS, nonsignificant,P>0.05; two-tailedPvalues for unpairedt-test. Bottom panels: CD25+, LAG-3+and CTLA4+T cells among 6.5 HA-specific or endogenous CD4+T cells on day 7 post infection. Full size image Figure 3: Impeded HA-specific CD4 + T-cell activation in the absence of IL-10 is not related to increased apoptosis or expanded regulatory T-cell populations. Naive WT or IL-10 KO HA-specific CD4 + T cells were adoptively transferred into WT or IL-10 KO mice, respectively, with 2.5 × 10 3 p.f.u. of influenza virus infection, as described in text. ( a ) CFSE staining profiles of HA-specific 6.5 CD4 + T cells on stated days post infection. HA-specific 6.5 CD4 + T cells adoptively transferred into naive mice without infection served as the control (grey shades). ( b ) Annexin-V staining of 6.5 + and endogenous CD4 + T cells in stated organs on day 7 post infection. ( c ) Regulatory T-cell populations. Top panels: Foxp3 + T cells among 6.5 HA-specific or endogenous CD4 + T cells on day 7 post infection. Values are mean±s.d. of at least three experiments; n =6; NS, nonsignificant, P >0.05; two-tailed P values for unpaired t -test. Bottom panels: CD25 + , LAG-3 + and CTLA4 + T cells among 6.5 HA-specific or endogenous CD4 + T cells on day 7 post infection. Full size image In the early phase of infection, IL-10 treatment enhanced the clonotypic expansion and the cytokine production of IL-10 KO HA-specific CD4 + T cells adoptively transferred into IL-10 KO mice. With supplemented IL-10 during the early phase of infection, daily from day 0 to day 3, the clonotypic percentage of HA-specific CD4 + T cells was increased from 1.48±0.4 to 3.64±0.3 in the lungs of the IL-10 KO adoptive transfer set. Production of IFN-γ and TNF-α by the IL-10 KO HA-specific CD4 + T cells was augmented as well ( Fig. 4 ). Supplemental IL-10 also caused increased clonotypic expansion (from 3.76±0.3% to 4.87±0.2%) and increased production of IFN-γ, TNF-α, and IL-10 by HA-specific CD4 + T cells in the lungs of the WT adoptive transfer set ( Fig. 4 ). Taken together, host IL-10 supports immune activation in the early phase of influenza virus infection. 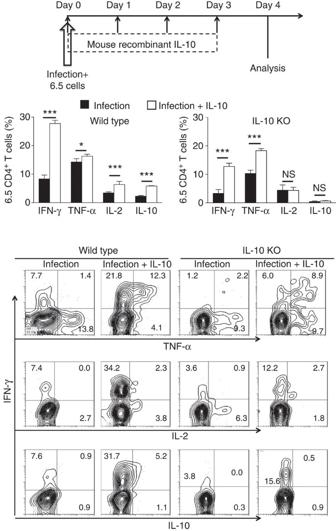Figure 4: Supplemental IL-10 facilitates Th1 cytokine production by influenza HA-specific CD4+T cells in the early phase of infection. Naive WT or IL-10 KO HA-specific CD4+T cells were adoptively transferred into WT or IL-10KO mice, respectively, with 2.5 × 103p.f.u. of influenza virus infection, as described in the text. Half of the mice of each group received intranasal supplemental recombinant mouse IL-10 daily for the first 4 days of infection. The other half of the mice received an equal volume of PBS and served as control. Cytokine production was analysed with 6.5 CD4+T cells from the lungs on day 4 post infection. Values are mean±s.d. of at least three experiments (n=6; ***P< 0.0001; *P< 0.01; NS, nonsignificant,P>0.05; two-tailedPvalues for unpairedt-test). Figure 4: Supplemental IL-10 facilitates Th1 cytokine production by influenza HA-specific CD4 + T cells in the early phase of infection. Naive WT or IL-10 KO HA-specific CD4 + T cells were adoptively transferred into WT or IL-10KO mice, respectively, with 2.5 × 10 3 p.f.u. of influenza virus infection, as described in the text. Half of the mice of each group received intranasal supplemental recombinant mouse IL-10 daily for the first 4 days of infection. The other half of the mice received an equal volume of PBS and served as control. Cytokine production was analysed with 6.5 CD4 + T cells from the lungs on day 4 post infection. Values are mean±s.d. of at least three experiments ( n =6; *** P < 0.0001; * P < 0.01; NS, nonsignificant, P >0.05; two-tailed P values for unpaired t -test). Full size image Early-phase Th1 evolution causes inflammation and disease Adoptive transfer experiments are often utilized to increase precursor frequency of antigen-specific T cells for in vivo studies of adaptive immunity. These experiments, such as ours with the HA-specific model system, are considered physiological [20] , [28] , [29] . However, increased antigen-specific T-cell precursor frequency may alter the disease. Therefore, we explored an influenza virus infection in IL-10 KO and WT mice without adoptive transfer. Without adoptive transfer of antigen-specific CD4 + T cells, IL-10 still supported T-cell activation in both IL-10 KO and WT mice. Compared with WT mice, IL-10 KO mice suffered from mild disease, with less weight loss and mortality ( Supplementary Fig. 4a ), despite unaltered viral kinetics of expansion and clearance ( Supplementary Fig. 4b ). There was less inflammation in the lungs of infected IL-10 KO mice, with reduced lymphocytes and plasma cell infiltration and less vasculitide changes ( Fig. 5a ). Proinflammatory cytokines IFN-γ and TNF-α were decreased in the lungs as well ( Fig. 5b ). With daily treatment of anti-IL-10 from day 0 to day 3 post infection, the early-phase IL-10 blockade attenuated the disease severity in infected WT mice ( Fig. 5c,d ) and reduced the proinflammatory cytokines IFN-γ and TNF-α in the lungs ( Fig. 5e ). In contrary, early-phase IL-10 supplements from day 0 to day 3 post infection aggravated disease severity in infected WT mice ( Fig. 5c–e ). These early-phase IL-10 modulations in the first 4 days of infection did not change the kinetics of viral clearance in the lungs ( Fig. 5f ). 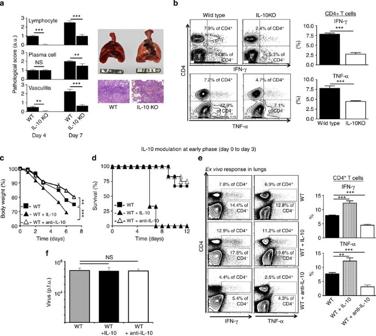Figure 5: IL-10 facilitated Th1 response leads to severe lung inflammation and disease in the early phase of influenza virus infection. WT and IL-10 KO mice were infected with 2.5 × 103p.f.u. of influenza virus. (a) Histopathological scores and gross pathology of the lungs on day 7 post infection. (b) Cytokine production in CD4+T cells of the lungs analysedex vivoon day 7. (c–f) Influenza virus-infected WT mice received recombinant mouse IL-10 or anti-IL-10 antibody daily for the first 4 days of infection. Mice were monitored for (c) body weight and (d) survival. (e) Cytokine production in CD4+T cells of the lungs was analysedex vivoon day 4. (f) Viral titres in the lungs were checked on day 4 post infection. Values are mean±s.d. of at least three experiments (n=6; ***P<0.0001; **P<0.001; NS, nonsignificant,P>0.05; two-tailedPvalues for unpairedt-test). Figure 5: IL-10 facilitated Th1 response leads to severe lung inflammation and disease in the early phase of influenza virus infection. WT and IL-10 KO mice were infected with 2.5 × 10 3 p.f.u. of influenza virus. ( a ) Histopathological scores and gross pathology of the lungs on day 7 post infection. ( b ) Cytokine production in CD4 + T cells of the lungs analysed ex vivo on day 7. ( c – f ) Influenza virus-infected WT mice received recombinant mouse IL-10 or anti-IL-10 antibody daily for the first 4 days of infection. Mice were monitored for ( c ) body weight and ( d ) survival. ( e ) Cytokine production in CD4 + T cells of the lungs was analysed ex vivo on day 4. ( f ) Viral titres in the lungs were checked on day 4 post infection. Values are mean±s.d. of at least three experiments ( n =6; *** P <0.0001; ** P <0.001; NS, nonsignificant, P >0.05; two-tailed P values for unpaired t -test). Full size image IL-10 suppresses HA-specific T cells in the absence of NA Splenocytes from naive WT or IL-10 KO 6.5 mice were stimulated in vitro. WT 6.5 HA-specific CD4 + T cells produced less IFN-γ and TNF-α compared with the IL-10 KO 6.5 cells upon overnight stimulation with cognate HA peptide or with PMA and ionomycin ( Fig. 6a ). IL-10 produced upon stimulation perhaps inhibited the cytokine production in the WT 6.5 cells ( Supplementary Fig. 5 ). However, WT 6.5 HA-specific CD4 + T cells produced more IFN-γ and TNF-α if stimulated overnight with influenza virus ( Fig. 6a ). The reverse trend was not altered back with further re-stimulation with cognate HA peptide or PMA+ionomycin ( Fig. 6b ). 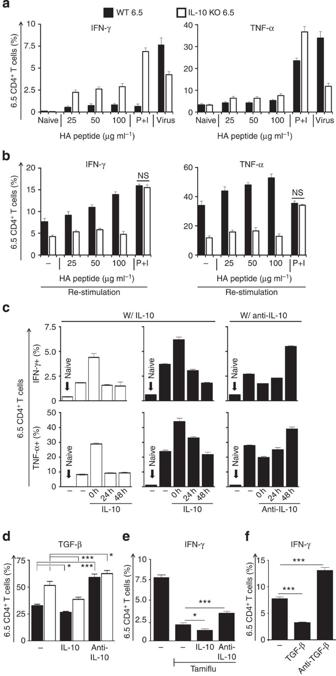Figure 6: IL-10 facilitates IFN-γ and TNF-α production by 6.5 HA-specific CD4+T cellsin vitroin the presence of viral NA or influenza virus. Splenocytes from naive WT or IL-10 KO 6.5 mice were stimulatedin vitro. (a) WT cells produced less IFN-γ and TNF-α than IL-10 KO cells upon overnight stimulation with HA peptide or PMA+ionomycin. However, WT cells produced more IFN-γ and TNF-α than IL-10 KO cells if stimulated overnight with influenza virus. Naive cells without stimulation served as control. (b) Influenza-stimulated WT cells produced more effector cytokines than the IL-10 KO counterparts even after further re-stimulation of cognate HA peptide or PMA+ionomycin. (c) Biphasic effect of IL-10 on IFN-γ and TNF-α production by 6.5 CD4+T cells in 72-h influenza virus coculture. IL-10 added at onset enhanced but IL-10 added at 48 h attenuated the production by both IL-10 KO (left panels) and WT cells (middle panels). In parallel, early-phase anti-IL-10 reduced but late-phase anti-IL-10 increased the cytokine production by WT cells (right panels). (d) Active TGF-β was elevated in IL-10 KO cells relative to WT 6.5 cells in overnight culture with influenza virus. IL-10 reduced and anti-IL-10 increased active TGF-β in 6.5 cells, if added at the onset of the culture. (e) With NA blockade, IL-10 suppressed and anti-IL-10 enhanced IFN-γ production in WT 6.5 cells, if added at the onset. (f) TGF-β inhibited and anti-TGF-β antibody enhanced the IFN-γ production by WT 6.5 cells, if added in the beginning. Values are mean±s.d. of at least three experiments in duplicates (***P< 0.0001; *P< 0.01; two-tailedPvalues for unpairedt-test). Figure 6: IL-10 facilitates IFN-γ and TNF-α production by 6.5 HA-specific CD4 + T cells in vitro in the presence of viral NA or influenza virus. Splenocytes from naive WT or IL-10 KO 6.5 mice were stimulated in vitro . ( a ) WT cells produced less IFN-γ and TNF-α than IL-10 KO cells upon overnight stimulation with HA peptide or PMA+ionomycin. However, WT cells produced more IFN-γ and TNF-α than IL-10 KO cells if stimulated overnight with influenza virus. Naive cells without stimulation served as control. ( b ) Influenza-stimulated WT cells produced more effector cytokines than the IL-10 KO counterparts even after further re-stimulation of cognate HA peptide or PMA+ionomycin. ( c ) Biphasic effect of IL-10 on IFN-γ and TNF-α production by 6.5 CD4 + T cells in 72-h influenza virus coculture. IL-10 added at onset enhanced but IL-10 added at 48 h attenuated the production by both IL-10 KO (left panels) and WT cells (middle panels). In parallel, early-phase anti-IL-10 reduced but late-phase anti-IL-10 increased the cytokine production by WT cells (right panels). ( d ) Active TGF-β was elevated in IL-10 KO cells relative to WT 6.5 cells in overnight culture with influenza virus. IL-10 reduced and anti-IL-10 increased active TGF-β in 6.5 cells, if added at the onset of the culture. ( e ) With NA blockade, IL-10 suppressed and anti-IL-10 enhanced IFN-γ production in WT 6.5 cells, if added at the onset. ( f ) TGF-β inhibited and anti-TGF-β antibody enhanced the IFN-γ production by WT 6.5 cells, if added in the beginning. Values are mean±s.d. of at least three experiments in duplicates (*** P < 0.0001; * P < 0.01; two-tailed P values for unpaired t -test). Full size image Exogenous IL-10 revealed a biphasic effect in the in vitro stimulation in the presence of influenza virus. When IL-10 was added at the beginning of the culture and HA-specific CD4 + T cells were analysed 72 h later, IFN-γ and TNF-α production by WT HA-specific CD4 + T cells was enhanced. The production was inhibited if IL-10 was added 48 h after the start of the culture ( Fig. 6c ). Anti-IL-10 antibody also revealed a biphasic effect, although in the opposite direction. Anti-IL-10 antibody added at the beginning of culture inhibited cytokine production, and cytokine production was enhanced if anti-IL-10 antibody was added 48 h after the start of the culture ( Fig. 6c ). IL-10 supported antigen-specific CD4 + T-cell activation in the presence of influenza virus. This support is associated with the viral NA activity during the early phase of culture. The desialylation with viral NA waned with time and there was only minimal desialylation on HA-specific CD4 + T cells after 48 h of culture (right panel, Supplementary Fig. 6a ). With reduced NA activity in the late phase, IL-10 reduced activation of antigen-specific CD4 + T cells. When influenza virus was added to the culture, viral NA caused desialylation on immune cells, including HA-specific CD4 + T cells. The desialylation was less apparent on WT than IL-10 KO HA-specific CD4 + T cells ( Supplementary Fig. 6a,b ). Accordingly, TGF-β activation was lower in the WT relative to the IL-10 KO HA-specific CD4 + T cells ( Fig. 6d ). The active TGF-β level was reduced with exogenous IL-10 and was increased with IL-10 blockade of anti-IL-10 antibody ( Fig. 6d ). IL-10 reduced activation in the early phase, even in the presence of influenza virus, if viral NA activity was blocked. IL-10 inhibited IFN-γ production by WT HA-specific CD4 + T cells in an overnight incubation cocultured with influenza virus, when the NA inhibitor Oseltamivir was added. Anti-IL-10 antibody reversed the suppressive effect of IL-10 on WT HA-specific CD4 + T cells ( Fig. 6e ). Viral NA induces the release of active TGF-β, a broad-spectrum immunosuppressive cytokine [30] . TGF-β should be the direct effector of immune suppression within the interplay between IL-10 and viral NA. Exogenous TGF-β inhibited and anti-TGF-β antibody enhanced the IFN-γ production by HA-specific CD4 + T cells in this in vitro system of overnight coculture with influenza virus ( Fig. 6f and Supplementary Fig. 7 ). With influenza virus infection in vivo , IL-10R expression on HA-specific CD4 + T cells increased as the viral NA activity in the lungs decreased after the first couple of days of infection. There were no significant differences between WT and IL-10 KO HA-specific CD4 + T cells ( Fig. 7a ). IL-10R remained upregulated until at least day 12 post infection. Supplemental IL-10 from day 4 to day 7 post infection impeded body weight loss and aided the recovery in infected WT mice ( Fig. 7b ). It is suggested that the upregulation of IL-10R is essential to pass immunoregulatory signals in humans and mice [31] , [32] , [33] , [34] , [35] . IL-10 imposed immune suppression as there was no substantial amount of viral NA and IL-10R that was upregulated. IL-10 blockade in this late phase of infection caused significant illness in WT mice and the mice eventually died ( Fig. 7b ). 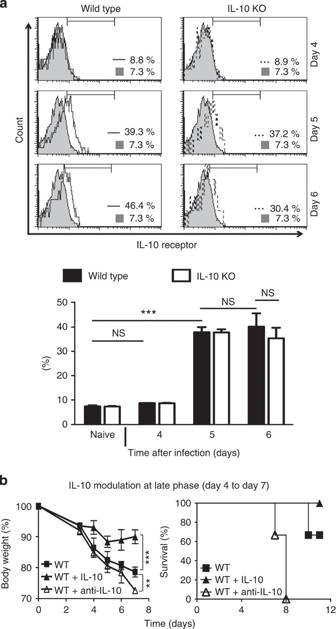Figure 7: IL-10Rs are upregulated and IL-10 attenuates body weight loss and helps in recovery during the late phase of influenza virus infection. (a) IL-10R was upregulated with time during influenza infection. Naive WT or IL-10 KO HA-specific CD4+T cells were adoptively transferred into WT or IL-10 KO mice, respectively, with 2.5 × 103p.f.u. of influenza virus infection. IL-10R on WT or IL-10KO HA-specific 6.5 CD4+T cells in the lungs were analysed on stated days post infection. HA-specific CD4+T cells adoptively transferred into naive mice without infection served as the control (grey shades). (b) IL-10 ameliorated the disease in the late phase of infection. WT mice received WT HA-specific CD4+T cells with 2.5 × 103p.f.u. of influenza virus infection and were divided into three groups. The first group received IL-10, second group received anti-IL-10 antibody and the third group received PBS daily for four consecutive days from day 4 post infection. Mice were monitored for body weight loss and survival. Values are mean±s.d. of at least three experiments (n=6; ***P< 0.0001; **P< 0.001; NS, nonsignificant,P>0.05; two-tailedPvalues for unpairedt-test). Figure 7: IL-10Rs are upregulated and IL-10 attenuates body weight loss and helps in recovery during the late phase of influenza virus infection. ( a ) IL-10R was upregulated with time during influenza infection. Naive WT or IL-10 KO HA-specific CD4 + T cells were adoptively transferred into WT or IL-10 KO mice, respectively, with 2.5 × 10 3 p.f.u. of influenza virus infection. IL-10R on WT or IL-10KO HA-specific 6.5 CD4 + T cells in the lungs were analysed on stated days post infection. HA-specific CD4 + T cells adoptively transferred into naive mice without infection served as the control (grey shades). ( b ) IL-10 ameliorated the disease in the late phase of infection. WT mice received WT HA-specific CD4 + T cells with 2.5 × 10 3 p.f.u. of influenza virus infection and were divided into three groups. The first group received IL-10, second group received anti-IL-10 antibody and the third group received PBS daily for four consecutive days from day 4 post infection. Mice were monitored for body weight loss and survival. Values are mean±s.d. of at least three experiments ( n =6; *** P < 0.0001; ** P < 0.001; NS, nonsignificant, P >0.05; two-tailed P values for unpaired t -test). Full size image IL-10 of HA-specific T cells facilitates their Th1 evolution We inoculated influenza virus into recipient mice with four adoptive transfer combinations to evaluate the relative significance of IL-10 from HA-specific Th1 cells versus IL-10 from cells other than the HA-specific T cells. IL-10 KO HA-specific CD4 + T cells were adoptively transferred into IL-10 KO or WT recipients, and WT HA-specific CD4 + T cells were adoptively transferred into IL-10KO or WT recipients. With IL-10 KO cells transferred into IL-10 KO recipients, the HA-specific CD4 + T cells responded with clonotypic expansion and production of Th1 cytokines IFN-γ, TNF-α and IL-2, all in total absence of IL-10 ( Fig. 8a ). The CD4 + T-cell responses were amplified with IL-10 from either the HA-specific CD4 + T cells or from other cells of the recipients ( Fig. 8a–c ). For facilitated clonotypic expansion and cytokine production by the HA-specific Th1 cells, IL-10 from HA-specific CD4 + T cell was relatively more important than the IL-10 from sources other than the CD4 + T cells. The enhancement was more obvious in the adoptive transfer set of WT HA-specific CD4 + T cells into IL-10 KO recipients than in the adoptive transfer set of IL-10 KO HA-specific CD4 + T cells into WT recipients ( Fig. 8a–c ). In all these adoptive transfer combinations, mice suffered from more severe disease with more IL-10 and the resultant more prominent Th1 responses ( Fig. 8d,e ). 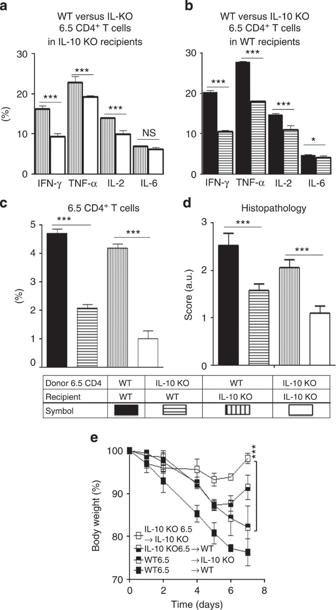Figure 8: IL-10 from HA-specific T cells facilitates their Th1 cytokine production. Adoptive transfer of naive 6.5 HA-specific CD4+T cells was performed in four combinations, with WT or IL-10 KO cells into WT or IL-10 KO recipients. The recipient mice were infected with 2.5 × 103p.f.u. of influenza virus and killed on day 7 post infection for analysis. (a) Cytokine production by WT or IL-10 KO 6.5 CD4+T cells in the lungs of IL-10 KO recipients; (b) cytokine production by WT or IL-10KO 6.5 CD4+T cells in the lungs of WT recipients; (c) 6.5 clonotypic percentages in the lungs; (d) lung pathology; and (e) body weight of the recipient mice, in the four adoptive transfer combination sets. Values are mean±s.d. (n=6; ***P<0.0001; *P< 0.05; NS, nonsignificant,P>0.05; two-tailedPvalues for unpairedt-test). Figure 8: IL-10 from HA-specific T cells facilitates their Th1 cytokine production. Adoptive transfer of naive 6.5 HA-specific CD4 + T cells was performed in four combinations, with WT or IL-10 KO cells into WT or IL-10 KO recipients. The recipient mice were infected with 2.5 × 10 3 p.f.u. of influenza virus and killed on day 7 post infection for analysis. ( a ) Cytokine production by WT or IL-10 KO 6.5 CD4 + T cells in the lungs of IL-10 KO recipients; ( b ) cytokine production by WT or IL-10KO 6.5 CD4 + T cells in the lungs of WT recipients; ( c ) 6.5 clonotypic percentages in the lungs; ( d ) lung pathology; and ( e ) body weight of the recipient mice, in the four adoptive transfer combination sets. Values are mean±s.d. ( n =6; *** P <0.0001; * P < 0.05; NS, nonsignificant, P >0.05; two-tailed P values for unpaired t -test). Full size image Our data revealed a correlation between Th1 cell-derived IL-10 and enhanced Th1 phenotype of HA-specific CD4 + T cells in the early phase of influenza virus infection. As IL-10 impedes NA activity and NA-induced activation of TGF-β, it is reasonable to suggest that IL-10 attenuates the release of activated TGF-β and counteracts the viral NA-mediated negative immune regulation in the early phase of infection. Suppressed negative immune regulation facilitates the Th1 evolution of influenza HA-specific CD4 + T cells. Facilitated Th1 activation with augmented IFN-γ, TNF-α and IL-2 production not only defends against infection but also causes inflammation and tissue injury. The influenza NA activity wanes with eradication of the virus. In the absence of abundant viral NA, IL-10 then preferentially binds to the IL-10R, which has been upregulated on HA-specific CD4 + T cells during the course of infection. IL-10 attenuates HA-specific CD4 + T-cell activation and curtails the inflammation to help recover from the illness in the late phase of infection. Although Th1 cells control their immune activity by IL-10 production, our data reveal a previously unexplored function of Th1-derived IL-10 in the early phase of influenza virus infection. Viral NA-mediated release of active TGF-β in the lungs during influenza virus infection was reported in 1996 (ref. 27 ). NA removes sialic acids on the LAP and the enzymatic cleavage causes the release of active TGF-β from its inactive precursor form [10] . TGF-β activation suppresses T-cell activation and implements invasion from the defensive immunity of the host. This has been reported in many parasitic, bacterial and fungal diseases [15] , [16] , [17] , [18] . TGF-β is a critical factor in our model of influenza virus infection and is related to the intensity of inflammation and the disease severity. It has also been reported that differential TGF-β activation by different NAs of various strains of influenza viruses is also critical for disease manifestations [10] . Increased TGF-β activity is correlated to better survival. TGF-β may be considered to be a target of immune modulation for severe influenza disease. The decisive evidence for IL-10 as an immunosuppressive cytokine is the phenotype of IL-10 KO mice. IL-10 KO mice develop chronic inflammatory bowel disease with age [32] . TGF-β KO mice develop a widespread multiorgan autoimmune disease [14] , one that is different than that of IL-10 KO mice. Transgenic mice with IL-10 overexpression demonstrate metaplasia of the mucous membrane with B and T cell-rich inflammation [36] . IL-10 increases IFN-γ, IFN-γ-inducible protein-10 and granzyme levels in healthy human volunteers [37] . There has been other evidence for the proinflammatory property of IL-10. IL-10 causes activation of B cells [38] , T cells [39] , [40] , natural killer cells [41] and mast cells [42] in mice. IL-10 blockade with anti-IL-10 antibody delays the onset of autoimmunity in mice as well [43] . It is uncertain whether IL-10 is indeed universally immunosuppressive. However, IL-10 suppresses immunity when IL-10 binds to IL-10Rs [31] , [34] , [35] , [44] . IL-10R expression on HA-specific CD4 + T cells remains at the base level in the early phase of our model of influenza virus infection. The IL-10R is composed of two subunits. The subunit IL-10R2 (IL-10Rβ) is constitutive and involved in downstream signalling [31] . The subunit IL-10R1 is inducible with stimulation and offers binding sites to IL-10 (ref. 31 ). IL-10R1 induction upregulates IL-10R expression, which is essential for IL-10-mediated suppression [31] , [34] , [35] . Ding et al . [44] demonstrated how IL-10R expression has a critical role in determining whether cells respond to IL-10. Perhaps the absence of upregulated IL-10R favours IL-10 interaction with the abundant viral NA in the early phase of influenza virus infection. IL-10 derived from the Th1 cells themselves is more effective in facilitating further Th1 evolution. This is possibly owing to the autocrine effect with geographic proximity of the cellular IL-10 and the viral NA-driven active TGF-β release on the same cell. The functions of immunity-related molecules are not always strictly black or white. Both pro- and anti- inflammatory properties have been described in literature for IL-17 (refs 45 , 46 ). The archetype proinflammatory mediator IFN-γ has been shown to have anti-inflammatory function as well [47] . We demonstrated LAG-3 as a suppressive molecule of regulatory T cells [28] at a time when LAG-3 had been believed to be an activation marker of Th1 cells [48] . Our finding has led to the exploration of anti-LAG-3 as a novel venue of cancer immunotherapy, targeting the abolishment of immune suppression mediated by LAG-3. The function of molecules such as these, including IL-10, may be pleotropic and may change, even in an opposite direction, as time evolves or other factors in the context deviate. The role of IL-10 in influenza virus infection is very difficult to study in humans. Translational research with experimental animal models is necessary. However, there are still barriers to the study of adaptive T-cell immunity in animal models. The precursor frequency of T cells with any antigen specificity is very low. With the adoptive transfer of HA antigen-specific CD4 + T cells, experiments in our transgenic mouse model revealed that IL-10 promotes inflammation and aggravates disease severity and mortality in the early phase of influenza infection. And yet, IL-10 curtails inflammation and ameliorates illness with improved survival in the late phase of infection. It is tempting to target IL-10 for immune modulation in severe disease of human influenza virus infection. However, as IL-10 is not necessarily totally immune suppressive, we have to be extremely cautious to avoid undesired effect and damage by an inappropriate manipulation of IL-10. Mice and influenza virus The Animal Care and Use Committee of the Chang Gung Memorial Hospital, Taiwan approved the animal use protocol (approval no. 2008092502). The committee recognizes that all the experiments involving the use of mice were carried out in strict accordance with the Animal Protection Law by the Council of Agriculture, Executive Yuan, Taiwan, ROC, and the guideline as shown in the guide for the Care and Use of Laboratory Animals as promulgated by the Institute of Laboratory Animal Resources, National Research Council. USA. All mice are of C57BL/10.D2 genetic background and 8–12-week-old mice of both sexes were used for experiments. The T-cell receptor (TCR) transgenic mouse line 6.5 expresses TCR recognizing an I-E d -restricted epitope 110 SFERFEIFPKE 120 of HA of PR8 influenza virus (generously provided by H. Von Boehmer, Harvard University, Boston, MA). The 6.5 mice were crossed with syngeneic IL-10 KO mice to generate 6.5 IL-10 KO transgenic mice. Syngeneic IL-10 KO mice were generated through breeding IL-10 KO mice of B10 genetic background (purchased from The Jackson Laboratories) onto C57BL/10.D2 genetic background for >9 generations. Mice were maintained in specific pathogen-free conditions. As IL-10 KO mice develop significant gut inflammation with age, even in pathogen-free conditions [32] , IL-10 KO or 6.5 IL-10 KO mice were used between 8–10 weeks of age, well before the onset of colitis. The PR8 (A/PR/8/34) strain of influenza virus was produced in the allantoic fluid of 10-day-old embryonated chicken eggs and characterized by a core facility at the Chang Gung University, Taiwan. Mice were inoculated via intranasal route during light diethyl ether anaesthesia (J.T. Baker, Phillipsburg, NJ) with indicated p.f.u of virus in 50 μl of PBS [20] . Administration of IL-10 and anti-IL-10 Recipient mice were intranasally infected with 2.5 × 10 3 p.f.u. of influenza virus on day 0. Mouse IL-10 (cat. no. I3019; Sigma Life Sciences) was administered intranasally during ether anaesthesia. For the early-phase modulation, IL-10 or anti-IL-10 (cat. no. I5145; Sigma Life Sciences) was given intranasally for the first 4 days of infection. Similarly, for late-phase modulation, IL-10 or anti-IL-10 was given intranasally from day 4 to day 7 post infection. Mice received 400 ng of IL-10 on the first day and 200 ng of IL-10 daily on the next three consecutive days of IL-10 modulation. Mice received 100 μg of anti-IL-10 antibody daily for four consecutive days. Control mice received equal volumes of the solvent (PBS) without anti-IL-10 antibody or IL-10. Adoptive transfer and CFSE staining Clonotypic HA-specific CD4 + TCR transgenic T cells were prepared from pooled spleen and lymph nodes of 6.5 transgenic mice. Similarly, clonotypic IL-10 KO HA-specific CD4 + TCR transgenic T cells were prepared from pooled spleen and lymph nodes of IL-10 KO 6.5 transgenic mice. Clonotypic percentage was determined by flow cytometric analysis. The naive phenotype was confirmed by profiles of activation markers CD44 and CD62L. 6.5 CD4 + T cells (2.5 × 10 6 ) were injected through the tail veins of the recipient mice in 0.2 ml of Hank’s balanced salt solution (HBSS). Clonotypic T cells (1 × 10 7 cells per ml) were stained with 5 μM of CFSE (5, 6-carboxyfluorescein diacetatesuccinimidyl ester; Molecular Probes, Eugene, Oregon) in HBSS for 10 min. Cells were washed three times with HBSS and CFSE-stained 6.5 CD4 + T cells (2.5 × 10 6 ) were transferred through the tail veins of the recipient mice. Flow cytometry Cell suspensions were incubated on ice with saturated concentrations of fluorochrome-labelled monoclonal antibodies in FACS buffer (PBS plus 0.5% bovine serum albumin and 0.02% NaN 3 ) as recommended by the manufacturers. Donor T cells were identified using mAbs: biotin conjugated anti-clonotypic 6.5 TCR (provided by H. Von Boehmer), avidin-Phycoerythrin (A1204, Caltag, Burlingame, CA) or streptavidin-APC (SA 1005, Caltag) and PerCP or fluorescein isothiocyanate (FITC)-conjugated anti-CD4 (553052 or 553047, BD Biosciences). Annexin-V binding buffer was used to stain Annexin-V (556420, BD Biosciences). All fluorochrome-conjugated antibodies were obtained from BD Biosciences except for T-bet, IgG1κ (45-5825, 45-4714, eBiosciences) and mature TGF-β (IC-1835A, R&D Systems). FITC- PNA (FL1071) was purchased from Vector Laboratories (Burlingame, CA). Cells were acquired on FACS CALIBUR and analysis was performed using CellQuest Pro (BD Biosciences) or FlowJo (Tree Star, Inc.) software. Intracellular cytokine staining Single-cell suspensions (5–10 × 10 6 cells per well in 24-well plates) from the harvested organs were re-stimulated for 5 h with 100 μg ml −1 major histocompatibility complex (MHC) class-II-restricted HA peptide ( 110 SFERFEIFPKE 120 ) in the presence of 5 μg ml −1 Brefeldin-A (Sigma-Aldrich). The concentration of Brefeldin-A was maintained throughout intracellular cytokine staining. Re-stimulated cells were surface stained with anti-6.5 and anti-CD4 as described above, fixed in intracellular fixation buffer (00-8222, eBiosciences), washed and stained in permeabilization buffer (00-8333, eBiosciences) containing fluorochrome-conjugated antibodies against target cytokines. For Foxp3 (11-5773, eBiosciences) and T-bet, cells were surface stained, fixed and permeabilized in fixation/permeabilization buffer (00-5523, eBiosciences), washed and stained in the permeabilization buffer (00-8333, eBiosciences) containing fluorochrome-conjugated antibodies. In some experiments, cells were analysed ex vivo and stained without re-stimulation. Plaque assay for virus titre We measured live influenza virus titre in the organs of infected mice using a modified Madin–Darby canine kidney cell (The American Type Culture Collection) plaque assay [20] . The organs were collected at the indicated times in 1 ml DMEM (Dulbecco’s modified Eagle’s medium), snap-frozen in liquid nitrogen and stored at −80 °C until analysed. Ten-fold dilutions of the tissue homogenates were prepared in DMEM supplemented with 10% FCS, antibiotic–antimycotic (15240-062, Gibco BRL), and 0.00025% Trypsin. A total of 500 μl of each dilution was added to confluent monolayers of Madin–Darby canine kidney cells in six-well plates and incubated for 1 h at 35 °C with 5% CO 2 . Each well of the culture received 2 ml of an agar overlay (0.3%) and was incubated for 3 days. Cells were fixed with 10% formalin, agar overlay was removed and fixed monolayers were stained by crystal violet (0.02% in 2% ethanol). The results were presented as p.f.u. per ml=(mean number of plaques × 2) × (each dilution factor). Histopathology The lungs from experimental mice were harvested on days as indicated and were fixed with 10% neutral-buffered formalin solution. Following fixation, the lungs were embedded in paraffin and 5-μm sections were cut. Sections were stained with haematoxylin and eosin and scored blindly. The infiltration of inflammatory cells, including lymphocytes, neutrophils and plasma cells, were separately scored by pathologist as negative, 1 + , 2 + or 3 + according to the density of infiltration. Vasculitis and fibrosis were also scored as negative, 1 + , 2 + or 3 + based on the severity [20] . Overall inflammation in the lungs was represented by the average of these scores. Cytokine production following in vitro stimulation Single-cell suspensions of splenocytes (5 × 10 6 cells per well) from naive WT or IL-10 KO 6.5 mice were stimulated in vitro . Splenocytes were cultured with different concentrations of cognate HA peptide (25, 50 or 100 μg ml −1 ) or PMA+ionomycin (10+250 ng ml −1 ). Brefeldin-A was added for last 5 h of stimulation and cells were then processed for intracellular staining without further re-stimulation. For overnight stimulation with influenza virus, splenocytes were cultured with influenza virus (PR8 strain; 0.1 multiplicity of infection (MOI)) in complete RPMI-1640. Cells were then processed for intracellular staining without re-stimulation or with stimulation of different concentrations of cognate HA peptide (25, 50 or 100 μg ml −1 ) or PMA+ionomycin (10+250 ng ml −1 ) in the presence of Brefeldin-A for 5 h. Naive cells without stimulation served as controls. For IL-10 or TGF-β modulation in influenza virus coculture, cells were cultured with influenza virus (PR8 strain; 0.1 MOI) for overnight or 72 h. IL-10 (10 ng ml −1 ), anti-IL-10 (20 μg ml −1 ), TGF-β (10 ng ml −1 , cat. no. GF346, Millipore), anti-TGF-β (10 μg ml −1 , cat. no. MAB1835, R&D) or Tamiflu (10 μg ml −1 , Roche) was added to the culture at the onset or at the stated time points. Cells were pulsed with 100 μg ml −1 HA peptide in presence of Brefeldin-A for the last 5 h of culture. NA activity on cell surface by PNA binding For in vitro NA activity, splenocytes (5 × 10 6 cells per well) from naive WT or IL-10 KO 6.5 mice were cocultured with influenza virus (0.1 MOI) overnight or for 48 h. Splenocytes without coculture with influenza virus served as control. Surface binding of FITC-PNA (FL1071, Vector Laboratories) to the mentioned cells was measured by flow cytometry. The in vivo NA activity was measured in the lungs of infected mice. WT or IL-10 KO 6.5 CD4 + T cells were adoptively transferred into syngeneic WT or IL-10 KO B10.D2-recipient mice, respectively, with 2.5 × 10 3 p.f.u. of influenza virus infection. Surface binding of FITC-PNA to the CD4 + T cells including 6.5 CD 4 + T cells from the lungs was analysed. Uninfected WT or IL-10 KO mice with adoptive transfer of WT or IL-10 KO 6.5 CD4 + T cells served as control. Chemical activity of mouse IL-10 in MUNANA-based NA assay The MUNANA (2′-(4-methylumbelliferyl)-α-D-N-acetylneuraminic acid) based NA assay is a standardized fluorescence-based assay and has been used for quantifying the chemical activity of NA. Viral or bacterial NA releases the fluorogenic end product 4-methylumbelliferone from the non-fluorescent substrate MUNANA by the enzymatic activity. The amount of released fluorescence directly relates to the amount of enzyme activity. MUNANA-based assays have been widely used in high-throughput screening for new NA inhibitors and influenza virus surveillance around the globe. We measured the effect of mouse IL-10 on NA activity by MUNANA-based NA assay in a 96-well plate. In brief, stated concentrations of mouse IL-10 in 10 μl of PBS (pH=7.2) were added to the 10 μl of 10 mM substrate in Tris-Cl (pH=7.2). Further, 2.5 × 10 3 p.f.u. of PR8 influenza virus in 10 μl of DMEM (pH=7.2) was added. An amount of 0.001 or 0.01 μg of neuraminic acid-A from S. pneumonia was used as positive control. The substrate with 10 μl of PBS and 10 μl of DMEM without NA or IL-10 served as the negative control. After 30 min of incubation, the plate was analysed for the fluorescence emitted by umbelliferone (355 nm/460 nm, 1.0 s). Release of active TGF-β by 6.5 CD4 + T cells WT or IL-10 KO 6.5 CD4 + T cells were adoptively transferred into syngeneic WT or IL-10 KO B10.D2-recipient mice. The 6.5 CD4 + T cells from the lungs and MLN were stained ex vivo with antibody against TGF-β1, β2 and β3 by intracellular staining on indicated days post infection. 6.5 CD4 + T cells from uninfected WT or IL-10 KO adoptive transfer sets served as control. On day 4 post infection, some of the harvested lung cells were stained ex vivo with antibody against TGF-β1, β2 and β3. Remaining lung cells were further cultured with recombinant mouse IL-10 (10 ng ml −1 ) or NA inhibitor Tamiflu (equivalent to 10 μg Oseltamivir per ml) in the presence or absence of influenza virus (0.1 MOI) for 5 h. The cells were then processed for intracellular staining of active TGF-β. Statistical analyses Data were represented as mean±s.d. We used GraphPad Prism version 5 for Student’s t -test analyses. We considered P values <0.05 as significant. How to cite this article: Dutta, A. et al . IL-10 inhibits neuraminidase-activated TGF-β and facilitates Th1 phenotype during early phase of infection. Nat. Commun. 6:6374 doi: 10.1038/ncomms7374 (2015).